Precise hierarchical self-assembly of multicompartment micelles Hierarchical self-assembly offers elegant and energy-efficient bottom-up strategies for the structuring of complex materials. For block copolymers, the last decade witnessed great progress in diversifying the structural complexity of solution-based assemblies into multicompartment micelles. However, a general understanding of what governs multicompartment micelle morphologies and polydispersity, and how to manipulate their hierarchical superstructures using straightforward concepts and readily accessible polymers remains unreached. Here we demonstrate how to create homogeneous multicompartment micelles with unprecedented structural control via the intermediate pre-assembly of subunits. This directed self-assembly leads to a step-wise reduction of the degree of conformational freedom and dynamics and avoids undesirable kinetic obstacles during the structure build-up. It yields a general concept for homogeneous populations of well-defined multicompartment micelles with precisely tunable patchiness, while using simple linear ABC triblock terpolymers. We further demonstrate control over the hierarchical step-growth polymerization of multicompartment micelles into micron-scale segmented supracolloidal polymers as an example of programmable mesoscale colloidal hierarchies via well-defined patchy nanoobjects. Nature fascinates with the rich functionality it creates from hierarchically self-organized complex architectures. The precision with which biology forms near monodisperse proteins or enzymes from polypeptides is unparalleled. In man-made self-assemblies, we pursue complex functional hierarchies with the ultimate goal to replace top-down approaches for the elegant and energy-efficient structuring of advanced materials [1] , [2] , [3] , [4] , [5] , [6] , [7] , [8] . Irrespective of the physical interaction used for achieving complex multilevel self-assemblies, there is an increasing bottleneck of precision engineering when constructing across length scales. The build-up of hierarchies requires control of the homogeneity of the subunits that order into the next higher level, as polydispersity can amplify throughout the process. With increasing size and complexity of the self-assembling building blocks, the kinetic obstacles become significant and trapping of metastable species can occur, preventing well-defined solution hierarchies of low polydispersity on an appropriate timescale [9] , [10] . Here, however, biology inspires a strategy to overcome this bottleneck as it teaches that the precise folding of peptides involves prefolded intermediates before furnishing monodisperse, perfectly functioning proteins or enzyme complexes. Thus, a step-wise restriction of the degrees of freedoms occurs [11] along a directional energy landscape, similar to a funnel ( Fig. 1 ) [12] , [13] . This calls for directing the self-assembly of synthetic bricks when increasingly complex hierarchical structures are targeted, especially when competing interactions and slow dynamics are involved. 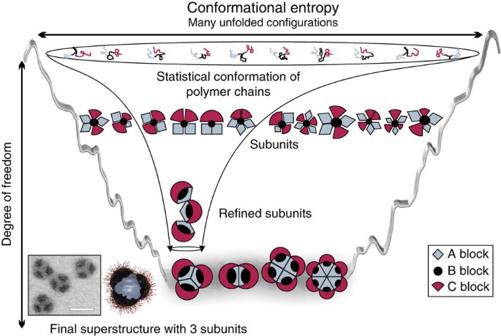Figure 1: Funnel concept for the directed hierarchical self-assembly of ABC triblock terpolymers in solution. Minimization of kinetic traps is realized by step-wise reduction of conformational freedom via pre-assembled subunits. In the first step, triblock terpolymers self-assemble into subunits, that is, pre-assembled intermediates, in a non-solvent for the middle block B (black), leaving different corona conformations of A (red) and C (grey). In the second step, the collapse of block A is triggered by exposure to a non-solvent for A and B, and higher-level assembly of the subunits occurs into the final superstructure. The process is accompanied by a refinement of the initial corona structure of A and C, and the conformational space narrows down into MCM superstructures of low polydispersity (Scale bar is 50 nm). Figure 1: Funnel concept for the directed hierarchical self-assembly of ABC triblock terpolymers in solution. Minimization of kinetic traps is realized by step-wise reduction of conformational freedom via pre-assembled subunits. In the first step, triblock terpolymers self-assemble into subunits, that is, pre-assembled intermediates, in a non-solvent for the middle block B (black), leaving different corona conformations of A (red) and C (grey). In the second step, the collapse of block A is triggered by exposure to a non-solvent for A and B, and higher-level assembly of the subunits occurs into the final superstructure. The process is accompanied by a refinement of the initial corona structure of A and C, and the conformational space narrows down into MCM superstructures of low polydispersity (Scale bar is 50 nm). Full size image In soft-matter nanotechnology, multicompartment micelles (MCMs) and their superstructures, formed by block copolymers, have emerged as a remarkable class of complex self-assemblies that allow to fundamentally understand the bottom-up structuring of solution-based hierarchies [14] , [15] , [16] , [17] , [18] , [19] , [20] , [21] , [22] , [23] , [24] , [25] , [26] , [27] , [28] , [29] , [30] , [31] , [32] . They are an intriguing class of responsive nanoobjects as they combine—similar to proteins—different physical nanoenvironments in well-segregated compartments and allow transporting different payloads simultaneously. Either the core or the corona can be compartmentalized, where we will concentrate on multicompartment-core micelles. We distinguish these further into spherical and linear MCMs, according to their geometric dimensions. Here, early studies reported on the formation of spherical MCMs with raspberry appearance formed by ABC triblock terpolymers, containing hydrocarbon, fluorocarbon and hydrophilic blocks. In recent years, Lodge and Hillmyer largely extended the space of morphologies by exploring the structures formed by ABC miktoarms in selective solvents, in which spherical MCMs, substructured vesicles and linear worm-like MCMs were identified [32] , [33] , [34] . Furthermore, the kinetically controlled (non-equilibrium) aggregation of solvent-swollen spherical micelles formed by ABC triblock terpolymers into linear substructured strands was achieved by complexation of the corona with oppositely charged complexing agents. Importantly, MCMs can bridge several length scales from segmented polymer chains (~10 nm) over substructured individual MCMs (25–100 nm) into extended superstructured cylinders (0.1–10 μm). So far, there has been best diversification of structures by promoting specific systems with non-linear polymer topologies or polymer-specific additives and processes [35] , [36] , [37] . However, looking at these systems, one can identify that it has remained challenging to establish a general concept, in particular for simple linear ABC triblock terpolymers, and more importantly, a scheme to predict and manipulate the architecture (patch distribution, geometry, linear versus spherical aggregates) of the resulting MCMs as a function of the polymer composition. For instance, football (aka raspberry) MCMs with various patches ( n ≈5–10) are the most common and also widely observed MCM morphology for triblock terpolymers [15] , [17] , [31] , [38] , [39] , [40] , [41] , [42] . However, it can be anticipated that there must be stable regions for MCMs possessing smaller amounts of patches (for example, 2,3,4) as such MCMs can be identified in polydisperse populations in present literature [31] , [35] , [36] , [43] , [44] . Consequently, the major question arises to how can these distinct patch numbers be obtained in high monodispersity? Also, what governs the aggregation into isolated spherical MCMs versus extended linear MCM strings? In the future, the self-assembly of block copolymers in solution will move to the second level of hierarchy, meaning that it becomes increasingly important to use MCMs as bricks to construct higher-level aggregates (second level), whereas present approaches mostly deal with the aggregation of block copolymers into micelles (MCMs, first level). Success in this direction however, critically depends on controlling patch distributions and achieving high monodispersity for MCMs so that they can serve as reliable bricks for the self-assembly into higher orders [23] . Here we demonstrate a general concept of what governs the amount of patches and how to achieve very homogeneous distributions of MCMs. Reasonably, only shallow differences in the free energy of MCMs with various patches can be expected and the challenge is to selectively target one specific morphology. Therefore, various MCMs in Fig. 1 are depicted on similar levels of free energy and we expect near-equilibrium structures when one is realized over the other. With the aim of avoiding undesirable kinetic traps, we take a different look at the structure formation and apply the concept of directed self-assembly by step-wise reduction of the degrees of freedom for the MCM formation of readily accessible linear ABC triblock terpolymers. This largely contrasts present approaches using one-step dissolution (or direct dialysis), and — as we will show — has a decisive influence on achieving superior control. Instead of considering MCMs as single entities with intact structures, we identify the essential pre-assembled subunits and target their formation in a dedicated first step. Using suitable solvents, we first construct well-defined micellar subunits with a collapsed but dynamic B core and a mixed or compartmentalized corona of blocks A/C (first reduction of conformational freedom). We chose to specifically direct the self-assembly via these intermediates as it assures the mechanistic pathway with high confidence and allows to sequentially reduce the dynamics from soluble to collapsed blocks. By lowering the solvent quality for block A, these subunits serve as bricks for the next-level assembly into various well-defined spherical MCMs with A core, B patches and C corona (second reduction of conformational freedom). This surprisingly simple step-wise approach allows maintaining significant dynamics for the subunits and directs the kinetic pathway during the self-assembly into unusually homogeneous MCMs. We regard this analogous to funnelling the structure formation along an energy landscape into final well-defined hierarchical architectures. With the aid of this approach, we demonstrate unique structural control over spherical MCMs. Moreover, we define conditions for which instead of spherical MCMs linear ones with alternating A and B segments will form via colloidal step-growth polymerization into mesoscale superstructures (colloidal polymers), as an example of colloidal LEGO based on well-defined patchy nanoobjects. This progress is accomplished with one of the simplest starting materials, that is, linear ABC triblock terpolymers, without the need of post-modifications or complexing agents. In combination with a herein developed scaling theory, we establish the stability criteria of different MCM morphologies and validate the general applicability by extending it to five types of terpolymers with widely different physical characteristics. Influence of volume ratio of core-forming blocks We start with a series of polystyrene- block -polybutadiene- block -poly(methyl methacrylate)s (PS- b -PB- b -PMMA; SBM1–12; Fig. 2 , Table 1 ), differing in the volume ratio of PS and PB blocks, V PS /V PB , and the molar ratio of coronal versus PS+PB units, r PMMA = N PMMA /( N PS + N PB ). We apply a two-step process for the directed self-assembly. The terpolymer is first dissolved in a non-solvent for the middle block PB, followed by dialysis into a non-solvent for both blocks PS and PB. Annealing of the subunits in the first solvent ensures near-equilibrium conformations at this stage. 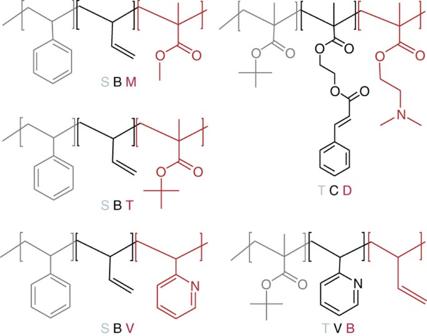Figure 2: Structures of the linear ABC triblock terpolymers. S, polystyrene; B, polybutadiene; M, poly(methyl methacrylate); T, poly(tert-butyl methacrylate; D, poly(2-(dimethylamino)ethyl methacrylate); V, poly(2-vinylpyridine); C, poly(2-(cinnamoyloxy)ethyl methacrylate). In each case, the red block builds up the corona. Figure 2: Structures of the linear ABC triblock terpolymers. S, polystyrene; B, polybutadiene; M, poly(methyl methacrylate); T, poly( tert -butyl methacrylate; D, poly(2-(dimethylamino)ethyl methacrylate); V, poly(2-vinylpyridine); C, poly(2-(cinnamoyloxy)ethyl methacrylate). In each case, the red block builds up the corona. Full size image Table 1 Molecular and micellar characteristics of employed ABC triblock terpolymers. Full size table Dissolution of SBMs in DMAc ( N,N -dimethylacetamide, non-solvent for PB, c= 1 g l −1 ) yields spherical micelles with a PB core and a mixed or compartmentalized corona of PS and PMMA, termed subunits. This is the first reduction of the degrees of conformational freedom in the directed self-assembly process. Dynamic light scattering (DLS) confirms their formation with small hydrodynamic radii of R h,app =9–14 nm ( Fig. 3a–c , Supplementary Fig. S1 and Table S1 ) [45] . In a second step, to direct the structure formation, dialysis against an acetone/isopropanol mixture (60/40 v/v) triggers the collapse of the PS block within the corona and induces higher-level aggregation of the subunits into the final multicompartment-core micelles (MCMs, Fig. 1 ). Rearrangements and phase segregation between PS and PMMA occur during this process, equalling a refinement of the subunits. Acetone is a non-solvent for PB, a near- Θ solvent for PS and a good solvent for PMMA. Isopropanol is a near- Θ solvent for PMMA and a non-solvent for both PS and PB. Hence, PB remains insoluble at all times, its chains yet mobile enough to allow for rearrangements during the process of subunit aggregation into the final MCMs. The importance of a dynamic PB core is underscored by the fact that freezing the segmental dynamics of the subunits via crosslinking the PB core results in ill-defined MCMs (see Supplementary Fig. S2 ). 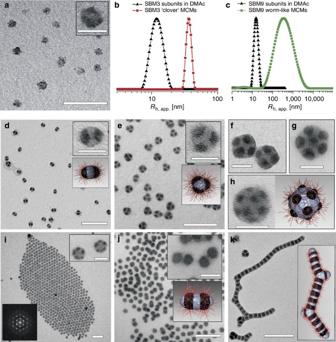Figure 3: Spherical and linear MCMs formed by SBMs with various core volume ratios (VPS/VPB). MCMs were prepared by dialysis of subunits with mixed- or compartmentalized PS/PMMA corona and PB core in DMAc into acetone/isopropanol (60/40 v/v). Staining was achieved with OsO4(PB black, PS grey, PMMA corona invisible). Subunits: (a) Weakly phase-segregated corona of PS and PMMA of SBM9 subunits with a PB core in DMAc. (b,c) DLS CONTIN plots of pre-assembled subunits and final MCMs of SBM3 and SBM9. MCMs: (d) SB2(BSB) 'hamburgers' of SBM6; (e) SB3'clovers' of SBM3; (f) SB4'Maltese crosses' of SBM4; (g) SB7'footballs' of SBM5; (h,i) SBx'footballs' of SBM1 and SBM2. The inset (lower right, i) depicts the Fourier transform of the TEM micrograph. (j) SBSBS=(SBS)2'double burgers' of SBM7 (see alsoSupplementary Fig. S3); (k) (SBS)xlinear MCM colloidal polymers of SBM9. The kinks in the colloidal polymers will be discussed below (Scale bars are 200 nm and 50 nm in the insets). Figure 3: Spherical and linear MCMs formed by SBMs with various core volume ratios ( V PS / V PB ). MCMs were prepared by dialysis of subunits with mixed- or compartmentalized PS/PMMA corona and PB core in DMAc into acetone/isopropanol (60/40 v/v). Staining was achieved with OsO 4 (PB black, PS grey, PMMA corona invisible). Subunits: ( a ) Weakly phase-segregated corona of PS and PMMA of SBM9 subunits with a PB core in DMAc. ( b , c ) DLS CONTIN plots of pre-assembled subunits and final MCMs of SBM3 and SBM9. MCMs: ( d ) SB 2 (BSB) 'hamburgers' of SBM6; ( e ) SB 3 'clovers' of SBM3; ( f ) SB 4 'Maltese crosses' of SBM4; ( g ) SB 7 'footballs' of SBM5; ( h , i ) SB x 'footballs' of SBM1 and SBM2. The inset (lower right, i) depicts the Fourier transform of the TEM micrograph. ( j ) SBSBS=(SBS) 2 'double burgers' of SBM7 (see also Supplementary Fig. S3 ); ( k ) (SBS) x linear MCM colloidal polymers of SBM9. The kinks in the colloidal polymers will be discussed below (Scale bars are 200 nm and 50 nm in the insets). Full size image Figures 3d–k depict transmission electron microscopy (TEM) micrographs of MCMs formed by various SBMs after OsO 4 staining (PS grey, PB black, PMMA invisible due to e-beam degradation). We observe spherical MCMs with PS core and distinct numbers (2–12) of PB patches for SBM1–6 ( Fig. 3d–i ). In contrast, SBM7–12 ( Fig. 3j,k ) show linear, partially segmented worm-like MCMs. The morphology (spherical versus linear) is determined by the volume ratio of the two insoluble blocks V PS /V PB . We find that SBM terpolymers with V PS /V PB >1 form spherical MCMs, whereas those with V PS /V PB ≤1 aggregate into linear MCMs. We will discuss the influence of the corona block later. In accordance to TEM, DLS confirms a 4-fold increase in hydrodynamic dimension for discrete spherical MCMs versus their preceding subunits ( Fig. 3b and Supplementary Fig. S1 ). For example, SBM3 subunits exhibit R h,app =11±2 nm in DMAc and R h,app =43±9 nm for the MCMs in acetone/isopropanol (60/40 v/v). Similarly, the radii dramatically increase to several μm for SBM7–12 caused by the progressing step-growth polymerization of micellar building blocks into segmented chains ( Fig. 3c ). The dominant population in SBM6 ( Fig. 3d ) are 'hamburgers' with a BSB core, which are different from SBM7 'double burgers' with an SBSBS=(SBS) 2 core sequence. Note the tendency of the 'double burgers' to undergo linear growth via end-to-end attachment in concentrated areas on the TEM grid ( Fig. 3j ). A detailed TEM grey-scale analysis in Supplementary Fig. S3 clearly reveals a step on each end of the 'double burger', which is absent for 'hamburgers', and confirms terminal PS compartments. These double burgers undergo step-growth polymerization into linear chains ( Fig. 3k ) for suitable corona volumes as will be shown below. From these experiments, we identify two key features. First, we generate a previously inaccessible diversity of well-defined MCM morphologies with remarkable control over the number of patches. Just using one simple triblock copolymer system, we are able to reproduce the established classes of MCMs, open pathways to rarely observed morphologies, such as 'clovers' [44] , and provide completely new core geometries like 'Maltese crosses' ( Fig. 3e,f ). Most importantly, we find homogeneous populations and not just single events among polydisperse mixtures [31] , [35] , [36] , [38] , [39] , [43] , [44] . This is significant, considering the delicate interplay of various thermodynamic factors and the shallow differences in free energy between the MCMs with various patches. For instance, SBM3 forms more than 92% 'clover' MCMs with 3 patches, whereas SBM6 forms above 90% 'hamburger' MCMs. Overall, the extent of controlled structure formation into homogeneous populations is unprecedented and a unique feature of our process. Secondly, in particular the spherical MCMs are not only homogeneous in number of patches but also remarkably monodisperse in size. This is evidenced by the formation of hexagonally ordered 2D lattices exhibiting third-order reflections in the corresponding Fourier-transformed image ( Fig. 3i ). The advantage of the herein developed directed self-assembly process with step-wise reduction of conformational freedom can be demonstrated by omitting the first dedicated reduction of conformational freedom (that is, the confinement into subunits). Common approaches to prepare MCMs include direct dissolution in the final solvent with very long equilibration times (days to weeks) [35] , [43] , [46] or one-step dialysis [15] , [39] . Direct dissolution of SBM into acetone/isopropanol only leads to polydisperse or even ill-defined aggregates for polymers with a large solvophobic fraction. During a single step, direct dialysis from a common solvent (THF), a pre-assembly into subunits can also take place but remains 'hidden' and uncontrolled while passing the various solvent compositions. On the one hand, this complicates an experimental analysis and mechanistic understanding. But, moreover, the final MCMs are also increasingly polydisperse and for large solvophobic fractions, meaning slower dynamics, only ill-defined agglomerates can be found. Detailed results on both are presented in Supplementary Figs S5,S6 and Supplementary Notes 1,2 . It may also be noted that our two-step process (dissolution in a non-solvent for PB, followed by dialysis) is similarly fast compared with direct dialysis and substantially faster and potentially more reliable than direct dissolution and prolonged equilibration. Consequently, clear advantages of the step-wise procedure can be identified in rapid preparation and the access to unique architectures with highly homogeneous populations. These advantages are most pronounced for systems containing large solvophobic/insoluble parts and, hence, slower dynamics. 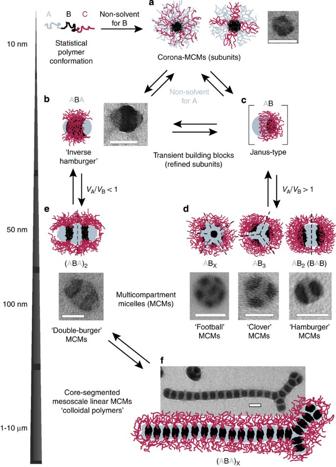Figure 4: Detailed mechanism for the preparation and directed hierarchical self-assembly of well-defined MCMs. First, the ABC triblock terpolymers are forced into (a) corona MCMs via dissolution in a non-solvent for B (termed subunits). Upon dialysis into a non-solvent for A and B, these subunits self-assemble further via a refinement of the corona structure (b,c) into various MCMs with well-defined number of patches (d,e). (f) Under suitable conditions, the colloidal polymerization into segmented worms can be triggered (TEM images, OsO4-stained; scale bars are 50 nm PS grey, PB black and PMMA not visible due to e-beam degradation). Detailed mechanism of directed self-assembly Figure 4 illustrates mechanistic details of the process. Here, we use the general ABC nomenclature as it applies to all triblock terpolymers. Dissolution in a non-solvent for B leads to micellar subunits ( Fig. 4a ). The extent of compartmentalization of the A and C corona depends on the interaction parameters between A and C and polymer/solvent [47] . Subsequent addition of a non-solvent for A induces its collapse. This collapse occurs slowly during the dialysis and leads to consecutive refinement of the A/C corona structure of the intermediate subunits ( Fig. 4b,c ) due to an enforced phase segregation of A and C. Rearrangements are allowed due to the dynamic B core. Classical core-shell-corona micelles are not observed under these conditions. At some point, the insufficiently swollen C blocks cannot stabilize the refining subunits anymore and secondary aggregation is triggered by the unfavourable exposure of solvophobic A patches. Consequently, initial subunits serve as building blocks for the MCMs ( Fig. 4d–f ). A transient AB Janus structure ( Fig. 4c ) is assumed during the merging of various subunits into spherical MCMs, thus forming distinct geometries. Figure 4: Detailed mechanism for the preparation and directed hierarchical self-assembly of well-defined MCMs. First, the ABC triblock terpolymers are forced into ( a ) corona MCMs via dissolution in a non-solvent for B (termed subunits). Upon dialysis into a non-solvent for A and B, these subunits self-assemble further via a refinement of the corona structure ( b , c ) into various MCMs with well-defined number of patches ( d , e ). ( f ) Under suitable conditions, the colloidal polymerization into segmented worms can be triggered (TEM images, OsO 4 -stained; scale bars are 50 nm PS grey, PB black and PMMA not visible due to e-beam degradation). Full size image Suitable polymers form 'inverse hamburger' ABA micelles with two A patches ( Fig. 4b ) under good solvent conditions for C and moderate solvent conditions for A. These are the crucial transient subunits for colloidal step-growth polymerization into linear 'double-burger' dimers ( Fig. 4e ), oligomers and colloidal polymers ( Fig. 4f ). They possess sticky terminal A compartments (if unprotected by an undersized corona), as the stabilizing corona chains only emerge from the non-terminal B patches. This supra-micellar polymerization of 'inverse hamburgers' via 'double burgers' into colloidal mesoscale chains is the soft-matter analogue to a recent approach for gold nanorods [48] . Scaling Theory We rationalize the thermodynamic stability criteria of MCM morphologies using the scaling approach, where we derive power law dependences for the MCM structures as a function of the degrees of polymerization, N A , N B , N C , of the segments and the solvent quality for the corona block C (see Supplementary Fig. S11 and Supplementary Note 3 for details). We start from micellar subunits with B core and A/C corona. Switching to poor solvent conditions for the A block induces its collapse. Two different scenarios of subunit aggregation are envisioned: strongly asymmetric, V A / V B ≫ 1, and nearly symmetric, V A / V B ≈1, core block volume ratios. For V A / V B ≫ 1, starlike or crew-cut spherical MCMs with n >1 B patches on the spherical A core are formed. A continuous B shell is instable when the interfacial tension between the solvophobic blocks becomes γ AB ≥ γ AS − γ BS , where S denotes the solvent. In the limiting case of starlike micelles ( d corana = R micelle − R core ≫ R core ) the number of patches, n , is Here, ℓ is the length of one monomer unit, τ C ≅ 1/2− χ CS quantifies the solvent strength for the coronal block C, ν A and ν B are the volumes of the corresponding monomer units and , where cosθ=( γ AS − γ AB )/ γ BS is the contact angle of B patches on the core. Since V A / V B >1, N B is neglected in equation (1b). In the limiting case of crew-cut MCMs ( d corona ≪ R core ), the number of patches is given by as long as the inter-patch distance h patch ≤ d corona . The experimental reality lies between these extremes. The number of B-patches, n , increases with V A / V B ≡ ν A N A / ν B N B and decreases with the solvent strength, τ C , and the length of the C block, N C . This theoretical prediction is in good agreement with our experimental results. For V A / V B ≈1 or V A / V B ≤1, the collapse of the A blocks only leads to a moderate increase in the overall solvophobicity of the terpolymers and, as a result, to a moderate growth of the (multicompartment) core. Aggregation of the micellar subunits into spherical MCMs ('hamburger', BAB) is not favoured ( Fig. 4 ). Gain in the overall interfacial energy promotes switching from BAB to ABA ('inverse hamburger', linear) favoured for where const is of the order of unity. When γ AS < γ BS , the core shape switching occurs at V A / V B >1. This leads to a stability region of ABA 'inverse hamburger', capable of linear polymerization. Considering the ABA 'inverse hamburgers' or the (ABA) 2 =ABABA 'double-burger' MCMs as monomers and dimers, respectively, for colloidal polymers, we estimate the number average degree of polymerization, as a mesoscale analogue to the chain-length distribution of supramolecular polymers or step-growth polymerization in synthetic polymers. A model for non-cooperative polymerization [49] yields: Here, c is the concentration and K denotes the equilibrium association constant between two MCMs, which depends on the excess free energy of one end of the worm-like MCM, E . K and E rise when decreasing the length or solvent quality for the corona, inducing longer supramicellar chains. Switching aggregate morphologies via corona volume As predicted by theory, the degree of subunit assembly of spherical and linear MCMs is also controlled by the corona volume (equations (1), (2) and (4)). This can be manipulated by the degree of polymerization of the C block, N C , or the solvent quality expressed by the excluded volume parameter, τ C ≅ 1/2− χ CS . The latter can also be elegantly tuned in stimuli-responsive corona blocks. Below, we demonstrate all of these possibilities. The basic reasoning is that a corona of insufficient expansion cannot effectively shield the underlying MCM subunits against aggregation via their exposed insoluble patches. 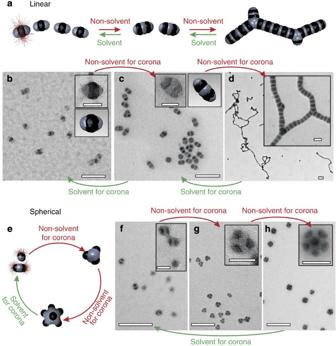Figure 5: Mesoscale polymerization of linear MCMs and subunit exchange of spherical MCMs promoted by changing the corona volume. The red corona chains emerge from the black compartments, but are mostly omitted for clarity (TEM images, OsO4-staining except (b) RuO4, acetone/isopropanol fractions are given in v/v). (a) Scheme for reversible mesoscale colloidal polymerization (SBM9). Note that the branching points are composed of (SBS)3centres. (b) SBS-refined subunits in acetone/isopropanol (90/10), (c) (SBS)2'double burgers' formed by two SBS in acetone/isopropanol (80/20) and their polymerization (d) in acetone/isopropanol (50/50). (e) Scheme for reversible exchange of refined subunits in spherical MCMs (SBM3). (f–h)In situswitching of spherical MCMs. (f) 'Hamburgers' and refined subunits successively merge into (g) 'clovers' and (h) 'footballs' triggered by reduction of the solvent quality for the corona (addition of isopropanol from 90/10 to 60/40 to 50/50). Refined subunits clearly reappear upon the expansion of the corona (addition of acetone from 50/50 to 90/10). Scale bars are 200 nm and 50 nm in insets. Figure 5 depicts the growth of linear (SBM9) and spherical (SBM3) MCMs by changing the solvent quality for the corona block. In DMAc, the initial subunits of SBM9 showed a weakly phase-separated PS/PMMA corona ( Fig. 3a ) [30] . Dialysis into acetone/isopropanol (90/10) induces a contraction of PS and a refinement of the structure as visible by the grey patches on the opposite sides of the PB core ( Fig. 5b ), that is, the formation of SBS 'inverse hamburger' MCMs (refined subunit). The increasing solvophobicity of the PS domains of these symmetrical building blocks and the concomitant contraction of the PMMA corona trigger the following dimerization and step-growth polymerization. Upon addition of further non-solvent (80/20) 'double-burger' dimers, (SBS) 2 , are formed as dominant species ( Fig. 5c ). A distribution of oligomers cannot be found here and thus we attribute their intermediate stability to a rearranged corona that is large enough to protect the terminal PS compartments, suppressing further growth (compare Fig. 4e ). At higher isopropanol content (70/30), slightly extended 1D oligomers are formed, followed by several μm long (60/40) and increasingly branched colloidal polymers (50/50; Fig. 5d ). Branches and kinks are caused by fusion/assembly of three SBS 'inverse hamburgers' into an (SBS) 3 branching point with one common PS domain in the centre. The drop in solvent quality contracts the corona and corresponds to an increase of the equilibrium association constant, K , as expressed in equation (4) and explains the formation of longer mesoscale colloidal polymers (DLS in Fig. 3c and Supplementary Fig. S4 ). Even higher isopropanol contents result in network formation and precipitation, caused by the increasing end-to-side addition, possible at stronger corona contraction. The polymerization is fully reversible by changing the solvent quality, for example, from 80/20 to 50/50 and back. Loosely related are results from Lodge and Hillmyer [43] who observed that addition of diblock copolymer micelles to MCM worms can induce a shortening of the worms via fusion/fission event. Figure 5: Mesoscale polymerization of linear MCMs and subunit exchange of spherical MCMs promoted by changing the corona volume. The red corona chains emerge from the black compartments, but are mostly omitted for clarity (TEM images, OsO 4 -staining except (b) RuO 4 , acetone/isopropanol fractions are given in v/v). ( a ) Scheme for reversible mesoscale colloidal polymerization (SBM9). Note that the branching points are composed of (SBS) 3 centres. ( b ) SBS-refined subunits in acetone/isopropanol (90/10), ( c ) (SBS) 2 'double burgers' formed by two SBS in acetone/isopropanol (80/20) and their polymerization ( d ) in acetone/isopropanol (50/50). ( e ) Scheme for reversible exchange of refined subunits in spherical MCMs (SBM3). ( f – h ) In situ switching of spherical MCMs. ( f ) 'Hamburgers' and refined subunits successively merge into ( g ) 'clovers' and ( h ) 'footballs' triggered by reduction of the solvent quality for the corona (addition of isopropanol from 90/10 to 60/40 to 50/50). Refined subunits clearly reappear upon the expansion of the corona (addition of acetone from 50/50 to 90/10). Scale bars are 200 nm and 50 nm in insets. Full size image The same principle of selective switching between high and low aggregation numbers can be applied to spherical MCMs (SBM3, Fig. 5e–h ). Decreasing the solvent quality for the corona block forces geometry changes into higher patch numbers and vice versa, in good accordance with theory. The process is fully reversible. Importantly, subunits, 'hamburgers', 'clovers' and 'football' MCMs show near identical average PB compartment sizes between 16.1±0.6 nm (evaluations given in Supplementary Fig. S7 ), thus supporting the exchange/release of intact refined subunits/individual patches. General validity of the concept In the last part, we demonstrate the general validity of our concept by applying it to vastly different block terpolymer systems. Those differ in: the selection of monomers, leading to different incompatibilities and solubilities; the polarity of the final solvent (dodecane/alcohols/water); the dynamics of the intermediate subunits as expressed by the bulk glass transition temperature, T g , of the middle block, varying from −51 to +100 °C. Furthermore, we exploit the stimuli responsiveness of a 'smart' polymer (PDMAEMA in TCD) to control colloidal superstructures by simply triggering a pH switch. Table 1 and Fig. 6 display the investigated terpolymers: SBV ( Fig. 6a ), SBT2 ( Fig. 6b ), TVB1 ( Fig. 6c ) and TCD ( Fig. 6d–f ) and also two polymers from our earlier work that conform to our concept ( t S f BT and N n BEO) [50] , [51] . 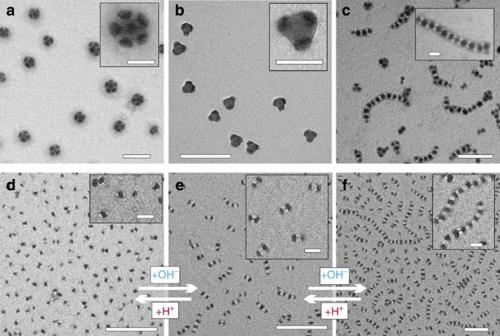Figure 6: MCMs of different triblock terpolymers. (TEM images, OsO4-stained if not mentioned otherwise; scale bars are 200 nm and 50 nm in insets). (a) SBV in acetone/isopropanol 20/80 (PB black, PS bright grey, P2VP corona grey). (b) SBT2 in ethanol (PB black, PS grey, PtBMA invisible due to e-beam degradation). (c) TVB1 in dodecane (I2staining; P2VP black, PtBMA white). (d–f) pH-programmable colloidal polymerization of TCD in water: (d) pH=3 completely protonated, (e) pH=6 partially protonated and (f) pH=10 deprotonated PDMAEMA corona (RuO4staining; PCEMA black, PtBMA bright grey, PDMAEMA corona not visible). Figure 6: MCMs of different triblock terpolymers. (TEM images, OsO 4 -stained if not mentioned otherwise; scale bars are 200 nm and 50 nm in insets). ( a ) SBV in acetone/isopropanol 20/80 (PB black, PS bright grey, P2VP corona grey). ( b ) SBT2 in ethanol (PB black, PS grey, P t BMA invisible due to e-beam degradation). ( c ) TVB1 in dodecane (I 2 staining; P2VP black, P t BMA white). ( d – f ) pH-programmable colloidal polymerization of TCD in water: ( d ) pH=3 completely protonated, ( e ) pH=6 partially protonated and ( f ) pH=10 deprotonated PDMAEMA corona (RuO 4 staining; PCEMA black, P t BMA bright grey, PDMAEMA corona not visible). Full size image Let us first change to different end blocks (C) and solvents, while keeping the same inner blocks. PS- block -PB- block -poly(2-vinylpyridine) (SBV) is dialysed from DMAc into isopropanol (selective solvent for P2VP) resulting in 86% 'hamburger' MCMs (see Supplementary Fig. S8 ). The large P2VP corona ( r P2VP =0.81) provides sufficient stabilization and the slightly asymmetric volume ratio ( V PS / V PB =1.67) favours spherical MCMs. As expected, a non-solvent for P2VP (addition of acetone to yield isopropanol/acetone 80/20) increases the degree of aggregation of subunits towards narrowly distributed 'football' MCMs ( Fig. 6a ). Next, PS- block -PB- block -( tert -butyl methacrylate) (SBT2) is dialysed from DMAc into ethanol (selective for P t BMA), leading to 'clover' MCMs ( Fig. 6b ), almost identical to SBM3, and in very good agreement with theoretical expectations, as SBT2 exhibits a comparable molar ratio of the corona units ( r P t BMA =0.32) and the same slightly asymmetric core volume ratio V PS /V PB =1.70. Furthermore, upon changing the composition to the range of SBM1/2, SBT1 exhibits 'football' MCMs (not shown here) due to a higher molar ratio of the corona units ( r P t BMA =0.67) and a strongly asymmetric core volume ratio V PS /V PB =8.23. The poly( tert -butyl methacrylate) -block -poly(2-vinylpyridine)- block -polybutadiene (TVB) series (see Table 1 ) broadens the concept to a completely new monomer sequence, very non-polar solvents and to a centre block with a much higher T g near 100 °C. The dialysis sequence from THF/cyclohexane (20/80; P2VP insoluble) to dodecane (selective for PB) yields linear MCMs ( Fig. 6c ). TVB1 forms extended linear structures due to the comparably small corona-forming block ( r PB =0.64). Branching in these mesoscopic worms occurs for higher ratios of V P t BMA /V P2VP (see Supplementary Figs S9,S10 ). Thus, even a high bulk glass transition temperature does not pose kinetic obstacles for the formation of well-defined MCMs in our step-wise process. Interestingly, all TVBs self-assemble into linear and branched MCMs despite their large core asymmetry ( V P t BMA /V P2VP >1), in apparent contrast to the other polymers. However, as derived in equation (3), the condition γ AS < γ BS , here γ P t BMA/S < γ P2VP/S , is fulfilled, that is, the surface tension of P2VP towards dodecane is higher as compared with P t BMA. Finally, the herein developed understanding enables us to command mesoscale micellar superstructures via a stimuli-responsive terpolymer, poly( tert -butyl methacrylate)- block -poly(2-(cinnamoyloxy)ethyl methacrylate)- block -poly(2-(dimethylamino)ethyl methacrylate) (TCD), in water. TCD has a high T g middle block and a pH- and temperature-sensitive, water-soluble PDMAEMA end block with p K a =6.2 (ref. 52 , Fig. 6d–f ). Micellar subunits are first formed in isopropanol, which is a non-solvent for PCEMA. Subsequent dialysis against water (pH=3) leads to TCT 'inverse hamburger' refined subunits ( Fig. 6d , V P t BMA /V PCEMA =1.17) stabilized by the fully protonated corona ( r PDMAEMA =0.62 in Table 1 underestimates its real extension). Next, we can exploit the smart corona to elegantly manipulate the colloidal self-assembly into linear MCMs, as the pH value regulates the corona swelling. At pH=6, the PDMAEMA corona is partially protonated, stretched and still occupies a moderately large volume. Hence, it provides good coverage of the compartmentalized core and 'double-burger' MCMs and linear oligomers are formed ( Fig. 6e ). At pH=10, the PDMAEMA corona is uncharged and contracted, thus inducing polymerization into extended linear mesoscale-MCM polymers ( Fig. 6f ). The pH-induced contraction of the PDMAEMA corona corresponds to an increase in the association constant K given in equation (4). This is a particularly elegant example of how to organize interactive polymer structures into nanostructured aggregates and harness their intelligent properties, as encoded via polymer chemistry, to control aggregation across several length scales, that is, from the polymer sequence to micrometer-long segmented worms. Such well-defined pH-programmable hierarchies drastically rely on highly defined colloidal building blocks of low polydispersity. We demonstrated the precise prediction of substructure, morphology, size and superstructures of self-assembled MCM hierarchies based on readily accessible linear triblock terpolymers. Therein, a directed step-wise self-assembly via pre-assembled subunits and sequential reductions of the degrees of freedom proved to be the key steps to reliably generate thermodynamically labile morphologies of MCMs with extremely homogeneous structure. This is not only expressed in the overall narrow size distribution but also manifests in a striking control over the number of patches. The latter is a substantial contribution and promising approach to the quest for well-defined patchy organic and inorganic nanoobjects [1] , [3] , [23] , [53] . In particular for low patch numbers, the resulting MCMs exhibit control of the geometry (angle and interpatch distance), wherein the dimensions can be tailored to potentially suit for sensing applications or the patterning of surfaces via nanolithographic procedures. For instance, the selective loading of patches with inorganics can lead to distinct spatial and tunable geometries of functional materials within ordered compartments. We also foresee that removal of the corona blocks (for example, when connected via supramolecular bonds) can be used to fabricate well-defined soft patchy nanoparticles not conceivable by other techniques. Interestingly, the switching of the geometries and patchiness of spherical MCMs, as well as the reversible aggregation of linear MCMs across length-scales during the step-growth polymerization from monomers into mesoscale chains, is enabled by the straightforward manipulation of the corona volume fraction. Such a high precision in structure and tunability contributes in satisfying the pressing need for homogeneous building blocks for the fabrication of future bottom-up materials. Our comprehensive development can be widely applied to other polymer systems and introduces a new paradigm for the design of polymer-based solution superstructures following surprisingly simple guidelines. Beyond that, our strategy answers the important challenge of how to induce selectivity in hierarchical structure formation of complex self-assemblies with wide conformational space and shallow energy landscape. Therefore, the discussed considerations of directing the self-assembly pathway with dedicated processes may well serve as inspiration for other self-assembling hierarchies, where large length scales with slow dynamics are approached and opens possibilities to overcome obstacles towards reliable structure formation therein. Looking out to the future, our understanding lays the cornerstones for the rational design of new generations of tunable and functional multicompartment solution-based hierarchies. Moreover, the accomplished comprehensive picture of the kinetics and pathways of MCM self-assembly into defined near-equilibrium structures establishes the necessary foundation for targeting defined non-equilibrium self-organized superstructures in the next steps. In consequence, the herein introduced concept paves the way for programmable particle hierarchies using anisotropic soft nanoobjects, where the balance of kinetics and thermodynamics can lead to new levels of complexity with superstructures also stable far from equilibrium. Materials The preparation and characterization of SBM, SBV, SBT and TVB triblock terpolymers were reported in detail previously [54] , [55] , [56] , [57] , [58] . Important parameters are summarized in Table 1 and Supplementary Table S1 . All solvents used were of analytical grade. Dialysis tubes of regenerated cellulose with a molecular weight cut-off of 12,000–14,000 g mol −1 were purchased from Roth, equilibrated in deionized water for 30 min and washed with excess dioxane before use. Preparation of subunits SBM, SBV and SBT terpolymers were dissolved in DMAc, TCD in isopropanol and TVB in a mixture of cyclohexane/THF (80/20 v/v). All polymer solutions were prepared at an initial concentration of 1 g l −1 . The as-prepared micellar solutions of SBM, SBV and SBT were annealed overnight at 70 °C, TCD and TVB at 50 °C to guarantee an equilibrated system. Afterwards, the resulting structures were investigated by both DLS and TEM. Self-assembly of MCMs In all cases, 5 ml of the micellar solution ( c =1 g l −1 ) were dialysed against 5 l of selective solvent for the corona block. The solvent exchange was monitored by 1 H-NMR. Micellar solutions of SBM terpolymers were dialysed against acetone/isopropanol mixtures, whereas in case of SBT terpolymer ethanol, and for SBV isopropanol (or an isopropanol/acetone mixture) was used. TCD was dialysed from isopropanol against water with pH values of 3, 6 and 10. TVB terpolymers were dialysed from cyclohexane/THF (80/20 v/v) mixtures into dodecane. For the determination of compartment size, size distribution and invariance of compartment size throughout assembly–disassembly steps, a quantity of at least 150 compartments were measured in TEM images, plotted as statistical histograms and evaluated to yield diameter distributions and average diameters. Dynamic light scattering DLS measurements were performed at a scattering angle of 90° or multiple angles ranging from 30° to 150° in 10° steps on an ALV DLS/SLS-SP 5022F equipment consisting of an ALV-SP 125 laser goniometer, an ALV 5000/E correlator and a He–Ne laser operating at a wavelength of λ =632.8 nm. The CONTIN algorithm was applied to analyse the obtained correlation functions. Apparent hydrodynamic radii were calculated according to the Stokes–Einstein equation. All CONTIN plots are intensity-weighted. Before the light scattering measurements, all sample solutions were filtered twice through a polytetrafluoroethylene filter with a pore size of 5 μm. The dynamic viscosities of acetone/isopropanol mixtures were calculated according to Ubbelohde, ,where ν is the kinematic viscosity, K is the viscometer constant, t is the measurement time, υ is the Hagenbach capillary correction factor, w 1 is the weight fraction of acetone and ρ i are the corresponding densities. Transmission electron microscopy TEM was performed in bright-field mode on Zeiss CEM 902 and LEO 922 OMEGA electron microscopes operated at 80 and 200 kV, respectively. The samples were prepared by placing one drop of the polymer solution (0.01 g l −1 ) onto carbon-coated copper grids. Excess solvent was instantly absorbed by a filter paper. For selective staining, the TEM specimens were exposed to RuO 4 vapour for 15 min (stains aromatics: PS, P2VP, PCEMA and partially PB), OsO 4 vapour for 2 h (stains double bonds: PB) or I 2 vapour for 4 h (stains amines: P2VP, PDMAEMA). How to cite this article: Gröschel, A. H. et al . Precise hierarchical self-assembly of multicompartment micelles. Nat. Commun. 3:710 doi: 10.1038/ncomms1707 (2012).